Loss ofGrem1-lineage chondrogenic progenitor cells causes osteoarthritis Osteoarthritis (OA) is characterised by an irreversible degeneration of articular cartilage. Here we show that the BMP-antagonist Gremlin 1 ( Grem1 ) marks a bipotent chondrogenic and osteogenic progenitor cell population within the articular surface. Notably, these progenitors are depleted by injury-induced OA and increasing age. OA is also caused by ablation of Grem1 cells in mice. Transcriptomic and functional analysis in mice found that articular surface Grem1 -lineage cells are dependent on Foxo1 and ablation of Foxo1 in Grem1 -lineage cells caused OA. FGFR3 signalling was confirmed as a promising therapeutic pathway by administration of pathway activator, FGF18, resulting in Grem1 -lineage chondrocyte progenitor cell proliferation, increased cartilage thickness and reduced OA. These findings suggest that OA, in part, is caused by mechanical, developmental or age-related attrition of Grem1 expressing articular cartilage progenitor cells. These cells, and the FGFR3 signalling pathway that sustains them, may be effective future targets for biological management of OA. OA causes a considerable global health burden, affecting 10 percent of people over the age of 60 [1] . OA affects all tissues of the joint including loss of AC, subchondral bone remodelling, osteophyte formation, synovial inflammation and joint capsule fibrosis, resulting in joint instability, pain and disability [2] . About 1 in 10 patients with knee OA will progress to joint replacement due to failure of medical care [3] . There is no cure for OA and existing treatments involve pain management and lifestyle modification [4] . There are several mouse models that induce OA via the surgical destabilization of medial meniscus (DMM) or collagenase-induced injury to destabilize tendons and ligaments (collagenase-induced OA, or CIOA). Articular cartilage (AC) is comprised of specialised chondrocytes that secrete a rich extracellular matrix (ECM) with high proteoglycan content, to allow effective movement between two bones [5] , [6] . Unlike growth plate (GP) cartilage, AC is a permanent tissue that requires the support of self-renewing progenitor cells to repopulate resident chondrocytes [5] , [7] , [8] , [9] , [10] , [11] . AC currently has limited regenerative capacity, with OA often resulting from injury, chronic mechanical stress or increasing age, with AC loss a key feature of OA [5] , [12] , [13] . Studies have confirmed skeletal stem cells [14] (SSC) based on immunophenotype [15] or lineage tracing [16] give rise to bone, cartilage and stroma but not fat lineages. Independently, a bone-fat (but not cartilage) progenitor cell population, marked by the expression of the Leptin Receptor ( Lepr ), was identified within the bone marrow [17] . The bone-cartilage-stromal progenitors in the growth plate and the bone-fat progenitors in the marrow express different markers ( Grem1 and Lepr , respectively) and have different roles during development and repair. Our initial study [16] focused on Grem1 -lineage tissue-resident SSCs in the GP of mice. A subsequent study found that tissue-resident SSC can be activated to make AC using microfractures in conjunction with BMP and VEGF signalling; however, the location of these AC-forming SSCs remained unknown, and these stimuli appeared to generate only cartilage, not subchondral bone [13] . Here, we show that a population of Grem1 -lineage chondrogenic progenitor (CP) cells, distinct from GP-resident SCCs, resides on the articular surface, and generates AC (and, in later stages, subchondral bone). We focus on the fate and function of these articular surface CP cells during aging, and upon OA-inducing injury using two independent models of OA (DMM and CIOA). We find that a Grem1 expressing CP Grem1 -lineage is lost through apoptosis in our OA models and that ablation of these CPs in young mice also causes OA. Single cell RNA sequencing (scRNAseq) of Grem1 -expressing cells at the articular surface reveals distinct molecular features of Grem1 -lineage cells and identifies FGFR3 signalling as a potential therapeutic target for Grem1 -lineage CP cell maintenance and expansion. The FGFR3 ligand, FGF18 (the active agent in Sprifermin) is currently in human clinical trial for OA treatment [18] . Injection of FGF18 into injured joints increases the number of Grem1 -lineage CP cells (but not mitosis in hypertrophic chondrocytes) and ameliorates OA pathology. Our study identifies a Grem1- expressing progenitor cell origin of articular cartilage, which is maintained, at least in part, by FGFR3 signalling, and when depleted results in OA. Grem1 CP cells are depleted in OA Focusing our studies on the knee joint of adult mice, we observed two anatomically distinct populations in the AC and GP marked by Grem1- lineage tracing (Fig. 1a ). Physically, these were separated in the femur by 800–1900 microns. Fig. 1: The articular Grem1 -lineage progenitor cells are significantly depleted in OA. a Representative image of knee joint from 8-week-old Grem1-TdT mice administered tamoxifen at 6 weeks of age showing the location of Grem1 cells in growth plate (GP), subchondral bone (SB) and articular cartilage (AC), n = 5 mice. b Experiment schema. DMM surgery was performed on adult Grem1-TdT , Acan-TdT and Lepr-TdT mice and tissue harvested after 8 weeks. c Representative image of proteoglycan loss, and d osteophyte-like formation (red dotted line) stained with Toluidine blue and Fast green in DMM with paired normal for comparison. n = 11 mice/group. e Representative images of paired distal femur joints of Grem1-TdT (top), Acan-TdT (middle) and Lepr-TdT (bottom) mice showing a decrease in Grem1 -lineage cells within the AC DMM injury site (arrows) compared to normal. f Quantification of Grem1 -, Acan - and Lepr -lineage cells as a percentage of total chondrocytes within the DMM injury site (filled circle) in comparison to no surgery (open circle) control. Grem1 and Lepr n = 4 animals/group, Acan n = 3 animals/group. Paired, two-tail t -test. g ColVII induced OA experiment schema. h Representative images of Grem1-TdT distal femur joints showing loss of Grem1 -lineage AC cells as indicated by arrows within the injury site (top), and OA pathology induced by ColVII compared to PBS control. Sections stained with Toluidine blue and Fast green, arrows indicate superficial lesions. i Quantification of the percentage of Grem1 -lineage AC cells per HPF (left) and, unblinded histopathological assessment using OARSI grading of OA pathology (right) in ColVII induced OA (square) compared to PBS controls (circle). n = 6 mice/group. Paired, two-tailed t test. j Representative images of TUNEL staining in articular Grem1 -lineage cells quantified in k . k Quantification of the number of articular Grem1 -lineage TUNEL positive cells in ColVII induced OA (square, n = 8 mice) compared to PBS control (circle, n = 7 mice). Unpaired, two-tailed t test. Bars denote s.e.m. Source data are provided as a Source Data file. Mouse image in figure schemas created with BioRender.com. Full size image OA is predisposed by injuries that destabilise the periarticular tissues of a joint [19] . We used two models of induced OA in mice, involving surgical DMM or collagenase VII degradation of intra-articular stabilising ligaments (CIOA), to examine the fate of Grem1 lineage cells, Lepr bone marrow derived-mesenchymal stem cells (MSC) and articular chondrocytes marked by Acan in OA. Rosa-TdTomato reporter mice crossed with Grem1-creERT , Acan-creERT and Lepr-cre (a constitutive Cre line), henceforth termed Grem1-TdT , Acan-TdT and Lepr-TdT mice respectively. These mice faithfully labelled Grem1- , Acan- and Lepr- cells and, depending on the time point following Cre mediated recombination of the reporter, their respective progeny. The inducible Cre lines, Acan-TdT and Grem1-TdT , were administered tamoxifen at 8 to 10 weeks of age, with DMM surgery (Fig. 1b , Supplementary Fig. 1a ) performed 2 weeks later. Lepr-TdT mice of similar age had DMM surgery for comparison (Fig. 1b ). DMM surgery results in a significant decrease in proliferating cells in both the superficial and non-calcified zones of the AC (Supplementary Fig. 1b ). OA pathology was confirmed by loss of proteoglycans, surface fibrillation (Fig. 1c ) and osteophyte formation (Fig. 1d ). Quantification of the total percentage of Acan , Grem1 and Lepr traced AC cells at the site of proteoglycan loss showed a significant decrease in the Grem1 -lineage population only (Fig. 1e, f ). This suggested Grem1 AC chondrocytes may be important in maintaining AC integrity and protection from daily mechanical insult. The absence of lineage-traced cells in the AC of Lepr-TdT mice is consistent with a prior study [17] and suggested that the primary role of the Lepr -lineage is in the haematopoietic niche in diaphyseal bone marrow [20] , [21] . Notably, the persistence of Acan AC chondrocytes in DMM animals suggests that the initial stage of OA is not due to total chondrocyte loss, but rather is specific to the loss of the Grem1 -lineage CP population. In the CIOA model (Fig. 1g ), we observed more severe OA pathology as expected [22] . As with DMM, Grem1-TdT CIOA mice exhibited significant loss of Grem1 -lineage CP cells through apoptosis, decreased AC thickness and increased OA pathology [23] compared to PBS injected animals (Fig. 1h–k , Supplementary Fig. 1c ). This suggested Grem1 -lineage articular surface CP cells may be important in the pathogenesis of OA. Grem1 marks a bipotent chondrogenic and osteogenic progenitor population in the AC Given that OA models were characterised by loss of Grem1 -lineage CP cells, we tested whether Grem1 -lineage CP cells were in fact resident stem-progenitor cells for normal articular cartilage post-natal development and maintenance. Grem1-TdT and Acan-TdT mice were administered tamoxifen at postnatal day 4 to 6 before sacrifice with age matched Lepr-TdT mice, to determine the contribution of each lineage to the AC (Fig. 2a ). Grem1 -lineage CP cells were immediately observed within the cartilaginous epiphysis and meniscus after a week, and had given rise to 39.4% of the AC. In later stages of development, we found the Grem1 -lineage CP cells also generated osteoblasts in subchondral bone, and by 1 month had populated the entire joint structure, including 30.7% of the AC (Fig. 2b ). A partially overlapping distribution of AC cells was observed with Acan progeny (Fig. 2b ). In contrast, Lepr -lineage cells [24] were not evident within the AC but were found as perisinusoidal cells in the bone marrow, consistent with a previous report [20] (Fig. 2b ). Immunofluorescence staining at 20 weeks (Fig. 2c and Supplementary Fig. 2a ) showed that Grem1 and Acan cells gave rise to SOX9+ and hypertrophic COLX+ chondrocytes, as well as OCN+ osteoblasts. In contrast, Lepr cells only gave rise to OCN+ osteoblasts, very occasional SOX9+ chondrocytes and no COLX+ chondrocytes (Fig. 2c , Supplementary Fig. 2a ). Fig. 2: Grem1 -lineage marks a progenitor cell population in the AC. a Experimental schema. b Representative images of AC from Grem1-TdT (top row) and Acan-TdT (middle row) mice and age paired Lepr-TdT (bottom row) mice. n = 5 animals per group per time point. c Distal femur from neonatal tamoxifen Grem1-TdT , Acan-TdT and Lepr-TdT pulse-chased for 20 weeks. Representative IF staining of Grem1 (top row), Acan (middle row) and Lepr (bottom row) cells expressing OCN, SOX9 and COLX (indicated by yellow arrows). Subchondral bone (SB), articular cartilage (AC) and meniscus (M). n = 3 mice per group. d Experimental schema. e Articular joints, outlined in yellow, were used to isolate red cells for in vitro assays. f Percentage of Grem1 -lineage (white) clones able to undergo expansion compared to Acan -lineage (grey) clones. g Number of CFU-F formed per clone. h , Representative images of Grem1 -lineage cells stained for CFU-F or differentiation markers Alizarin Red (osteo), Alcian blue (chondro) and Oil Red O (adipo). i Number of Grem1 - (white) or Acan -lineage (grey) clones that had undergone differentiation quantified as % of the total number of clones. f – i cells pooled from n = 3 animals, 22 clones per lineage. j Experimental Schema (right). Quantification of the total number of Grem1 -lineage cells within the superficial and calcified zones as a percentage of the total number of chondrocytes within the AC at 8 weeks (filled circle, n = 4 mice), 10 weeks (square, n = 3 mice), 18 weeks (triangle, n = 4 mice), 32 weeks (diamond, n = 4 mice) and 58 weeks (open circle, n = 4 mice) of age (left). Bars show s.e.m. k Representative images of adult articular joint showing H&E of zonal organisation of chondrocytes in the superficial zone (SZ), non-calcified zone (NCZ) and calcified zone (CZ) and Grem1 -lineage AC cells moving towards the CZ from 8 weeks (middle) to 32 weeks (right) of age. Superficial chondrocytes indicated with yellow arrows. f , i Two-sided Fisher’s exact test. g Two-sided unpaired t test. j Two-way Anova Tukey’s test. Bars denote s.e.m. Source data are provided as a Source Data file. Mouse image in figure schemas created with BioRender.com. Full size image To further analyse the clonogenic and differentiation potential of Grem1 -lineage CP cells in the early adult knee ex vivo, Grem1-TdT and Acan-TdT mice were administered tamoxifen at 6 weeks of age and knee joints harvested 2 weeks later (Fig. 2d ). Grem1 labelled specific articular surface cells (Fig. 2e ) overlapping with, but more limited than, the total Acan chondrocyte population (Supplementary Fig. 2b ). These Grem1- and Acan- traced cells from the AC of the tibiofemoral joint were isolated via flow cytometry and plated at clonal density (Fig. 2e ). As Lepr cells were not found in the AC (Supplementary Fig. 2c ), a Lepr comparable population could not be included in this AC-specific experiment. Grem1 -lineage articular CP clones were more frequently capable of serial propagation, in contrast to Acan clones (Fig. 2f ). Furthermore, Grem1 expression was significantly higher in Acan clones capable of in vitro expansion compared to those that were not (Supplementary Fig. 2d ), suggesting Grem1 expression correlated with self-renewal in vitro. Of the Grem1- and Acan- lineage clones that underwent >3 passages, no significant difference in CFU-F efficiency was observed (Fig. 2g ). When subjected to multilineage differentiation, both adult Grem1- and Acan- lineage clones gave rise to osteogenic (alizarin red stain+) and chondrogenic (alcian blue stain+), but not adipogenic (oil red O stain+) progeny (Fig. 2h , Supplementary Fig. 2e ). This is consistent with previous studies on postnatal whole bone populations [16] . A significantly greater percentage of Grem1 -lineage clones were capable of osteogenic differentiation compared to Acan -lineage clones (100% vs 25%, <0.0001, Fig. 2i ). Normal AC development and maintenance requires both interstitial and appositional growth of the AC [7] . Using long-term cell fate tracing of adult Grem1 -lineage cells in vivo, these cells contributed to progenitor populations in the superficial zone of the AC and with a significant increase in the percentage of Grem1 -lineage cells within the calcified zone of the AC with age (Fig. 2j, k ). Grem1 -lineage articular CP cells are lost with age To measure the longevity of Grem1 lineage cells within the tibiofemoral joint, 6-week-old Grem1-TdT mice were administered tamoxifen in early adulthood and analysed during aging (Fig. 3a ). There was a significant decrease in Grem1 -lineage articular CP cells from young to aged adult mice (Fig. 3a, b ). This is consistent with other studies looking at the presence and regenerative capacity of skeletal stem cells in aged animals [13] , [25] . The reduced regenerative capacity of the AC with age is due, at least in part, to reduced Grem1 -lineage articular CP cells and chondrocyte proliferation (Supplementary Fig. 3a, b ). Fig. 3: Grem1 -lineage articular progenitors cells are lost with age and targeted ablation causes OA. a Experimental schema. Quantification of total Grem1 -lineage articular chondrocytes (AC) as a % of the total ACs. n = 4 animals per time point, except 10wk n = 3. One-way Anova Tukey’s test. b Representative images of the Grem1-TdT articular knee joint from a . c Schematic of the Grem1-Td-DTR knock-in construct (top) and experimental outline. d Representative images of early adult mice articular joints treated with PBS or DT stained with anti-RFP. e Quantification of Grem1 AC cells as a % of the total number of AC chondrocytes in PBS (blue, n = 4 mice) or DT treated (red, n = 7 mice) Grem1-Td-DTR mice. Two-tailed Welch’s t test. f Representative images of ColX staining of Grem1-Td-DTR joints from WT and HOM DT-treated animals, n = 3 mice/group. Boxed regions indicate loss of ColX chondrocytes following ablation of Grem1 -expressing articular cells in HOM DT treated mice. g Representative image of DT treated articular joint of Grem1-Td-DTR mice ( n = 7 mice) stained with Tol blue and fast green showing pathological changes commonly associated with OA including AC damage indicated by red arrows, h loss of proteoglycan in the AC indicated by yellow arrows, i hypertrophic chondrocytes, j SB invasion, and k meniscus pathology. l Blinded scoring of average OA score following 3 days DT treatment in control wild-type mice (WT-DT, n = 9 mice), homozygous Grem1-Td-DTR mice (HOM-DT, n = 7) or PBS Grem1-Td-DTR mice (HOM-PBS, n = 4). One-way Anova Tukey’s test. m Single cell RNA (scRNA) sequencing experiment schema for isolation of Grem1 -lineage articular cells from mouse knee and analysis to show high Grem1 (red) , high Acan (blue) or high both Grem1/Acan expressing (magenta) populations. Bars denote s.e.m. Source data are provided as a Source Data file. Mouse image in figure schemas created with BioRender.com. Full size image We next examined whether Grem1 -lineage CP cells persist in the aging knee by administration of tamoxifen to Grem1-TdT mice at 29 weeks-of-age, in comparison to postnatal (week 1) or early adulthood (6 weeks), and visualisation of lineage traced cells 2 weeks later (Supplementary Fig. 3c ). Grem1 -lineage cell number decreased significantly with increasing adult age, with only <0.4% of total articular surface cells being Grem1 -lineage cells in early middle-age (Supplementary Fig. 3d, e ). At this stage, Grem1 -lineage cells were mainly observed in the subchondral marrow space and occasionally in the retained, but no longer proliferating GP (Supplementary Fig. 3f ). Targeted ablation of Grem1 articular CP cells causes OA The previous experiments confirmed that Grem1- lineage AC resident cells are bipotent chondro-osteogenic progenitor cells. To functionally test whether ablation interrupts the development of the AC we generated a new knock-in mouse line and employed other genetic ablation experiments. We had previously examined the role of Grem1 -lineage cells in postnatal skeletogenesis using a diphtheria toxin ablation model ( Grem1 - creERT;R26-LSL-ZsGreen;R26-LSL-DTA ), in which the Grem1 -lineage was incompletely ablated [16] . Nevertheless, post-natal ablation of Grem1 -lineage cells led to significantly reduced femoral bone volume by microCT after two weeks, with reduced trabecular bone as quantified by histology [16] . To achieve more complete ablation of Grem1 -expressing cells, we generated a new Grem1-DTR-TdTomato knock in mouse model ( Grem1-DTR-Td) in which Grem1 actively expressing cells concomitantly express the TdTomato reporter and the Diphtheria toxin receptor (DTR), rendering these cells susceptible to diphtheria toxin (DT) ablation (Supplementary Fig. 3g ). Grem1-DTR-Td mice were administered 2 doses of DT intra-articularly, to target the articular population of Grem1- expressing cells, at 5 to 6 weeks of age and the mice were sacrificed 3 days later (Fig. 3c ). This induced a significant reduction in Grem1 CP cell number in the AC but not GP, increased COLX+ articular chondrocytes and induced OA pathological changes compared to age-matched controls (Fig. 3d–l , Supplementary Fig. 3h, i ). The worsening in OA pathology scoring in the Grem1 -cell ablation group was predominantly due to cartilage hypertrophy, proteoglycan loss and structural damage, with a lesser contribution from meniscus pathology and subchondral vascular invasion and zero scoring from subchondral bone sclerosis or osteophyte changes. To confirm the role of adult Grem1 CP cells in OA, we utilised a second transgenic mouse model of targeted cell ablation generated by mating Grem1-TdT mice to Rosa-iDTR mice to create Grem1-TdTomato-iDTR mice ( Grem1-creERT;DTR) . DTR expression on Grem1 -lineage cells was induced by tamoxifen administration at 4 weeks of age, followed by local ablation of Grem1 -lineage AC cells by intra-articular injection of DT at 8-weeks-old for 2 weeks, before animals were sacrificed at 26 weeks (Supplementary Fig. 3j ). Analysis of OA pathology and quantification of Grem1 -lineage articular surface CP cells showed a significant loss in Grem1 -lineage AC cells concomitant with worsened OA pathology, including a reduction in AC thickness (Supplementary Fig. 3k ). Together our data confirmed that Grem1 -expressing CP cells are normal progenitor cells that are lost in aging and in mechanical trauma-mediated OA and their depletion directly results in OA. While we showed that loss of Grem1 -expressing CP cells is an early event in OA (Fig. 1 ) and, in turn, also causes OA (Fig. 3 and Supplementary Fig. 3 ), we considered the possibility that OA may also be caused, in part, by the death or degeneration of the resultant Grem1- lineage, mature Acan -expressing chondrocytes. To first understand the degree by which Grem1 -lineage CPs may be distinct from Acan- expressing articular chondrocytes, we undertook scRNAseq transcriptomic analysis of FACS-isolated single cells from early adult Grem1-TdT knee AC following tamoxifen administration (Fig. 3m ). This analysis showed that while the majority (72%) of these Grem1 -lineage traced cells expressed Acan , we could also identify Grem1 -lineage cells that did not express Acan (Fig. 3m ). This was consistent with co-immunofluoresence staining of knee sections in which double positive Grem1 -lineage/ACAN+ cells were observed in the articular cartilage, but also discrete Grem1 -lineage and ACAN expressing populations (Supplementary Fig. 3l ). To investigate potential differences between Grem1 and Acan expressing AC cells, we identified significantly differentially regulated transcripts between Grem1 + Acan- and Grem1-Acan + populations in our scRNAseq dataset (Supplementary Fig. 3m ). The most highly upregulated transcript in Grem1 + Acan- compared to Grem1-Acan + populations was Islet1 (Isl1 ). Isl1 encodes an essential LIM-homeodomain transcription factor important for progenitor populations and differentiation across multiple tissues including islet cells and pancreatic mesenchyme [26] , motor neurons [27] and cardiovascular progenitor populations [28] , but with an underexplored potential function in the AC. Together with differential expression of genes with roles in cartilage or arthritis, such as platelet derived growth factor receptor alpha ( Pdgfra , [29] ), procollagen C-endopeptidase enhancer 2 ( Pcolce2 , [30] ) and hyaluronan and proteoglycan link protein 1 ( Hapln1 , [31] ), we noted reduced expression of three collagen transcripts ( Col9a2, Col9a3, Col27a1 ) in the Grem1 + Acan- compared to Grem1-Acan + populations (Supplementary Fig. 3n ). These transcripts encode key components of the type IX and XXVII extracellular matrix collagens, with vital roles in skeletal and cartilage development in mice and humans [32] , [33] , [34] . Altogether, this analysis suggested that Grem1 -expressing articular CPs overlap with the broader Acan -expressing population, but are also distinct, and may have distinct functionality generated by differential expression of genes important for cartilage and progenitor populations. Previous studies noted that ablation of chondrocytes marked by Acan or Prg4 results in mild OA that resolves over time, or no OA [35] , [36] . To further discriminate the role of Acan+ chondrocytes in comparison to Grem1 -lineage CPs in OA, we compared the OA phenotype caused by ablation of each cell population using similar genetic models and induction regimens. DT treatment of Acan-creERT;DTR mice caused a significant decrease in ACAN-expressing cells, and a mild but significant increase in OA pathology scoring at 26 weeks in comparison to PBS treated controls (Supplementary Fig. 3o, p ). The overall average OA score in Acan -lineage ablated mice was 0.53 (+/− 0.27, st.dev.) in comparison to 1.75 (+/− 0.68) in the Grem1-TdT-DTR mice treated with DT (Supplementary Fig. 3k, o, p ). These data are consistent with previous Acan- and Prg4- chondrocyte ablation experiments reported to generate mild or insignificant OA [35] , [36] . Given these differences, we note that OA is not just a disease of mature chondrocyte loss, but is likely also a failure of local progenitor regeneration. We next used flow cytometry to isolate Grem1 -lineage cells from early adult mice and implanted them into recipient mice that had undergone DMM surgery via intra-articular injection (Supplementary Fig. 3q ). This initial effort to implant Grem1 -lineage cells was hindered by inefficient homing to and/or survival of the cells in the AC (Supplementary Fig. 3r ). Thus, we subsequently studied how to preserve this important population through normal aging (Fig. 3 ) or injury associated (Fig. 1 ) attrition that could be key for OA prevention. Grem1- lineage single cell transcriptomics revealed a distinct population of articular chondrocytes We applied scRNAseq analysis to characterise FACS-isolated early adult Grem1 -lineage CP cells from the epiphysis proximal to the GP and compared to Grem1 -lineage cells within the GP, as well as age-matched skeletal cells defined by the Lepr lineage (Supplementary Fig. 4a, b ). Unsupervised clustering of our pooled scRNAseq data revealed 6 distinct cell clusters: five Grem1 -lineage (AC1-2, GP1-3) and one Lepr cluster (Fig. 4a, b , Supplementary Fig. 4c–e ). Though there were substantial similarities in transcript expression in the articular surface and GP cells, clusters within the Grem1 -lineage cells in the articular surface could also be separated by differential transcript expression from those in the GP (Fig. 4a, b , Supplementary Fig. 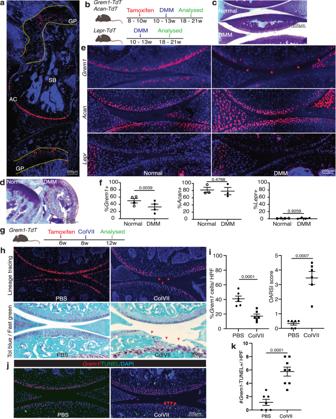Fig. 1: The articularGrem1-lineage progenitor cells are significantly depleted in OA. aRepresentative image of knee joint from 8-week-oldGrem1-TdTmice administered tamoxifen at 6 weeks of age showing the location ofGrem1cells in growth plate (GP), subchondral bone (SB) and articular cartilage (AC),n= 5 mice.bExperiment schema. DMM surgery was performed on adultGrem1-TdT,Acan-TdTandLepr-TdTmice and tissue harvested after 8 weeks.cRepresentative image of proteoglycan loss, anddosteophyte-like formation (red dotted line) stained with Toluidine blue and Fast green in DMM with paired normal for comparison.n= 11 mice/group.eRepresentative images of paired distal femur joints ofGrem1-TdT(top),Acan-TdT(middle) andLepr-TdT(bottom) mice showing a decrease inGrem1-lineage cells within the AC DMM injury site (arrows) compared to normal.fQuantification ofGrem1-,Acan- andLepr-lineage cells as a percentage of total chondrocytes within the DMM injury site (filled circle) in comparison to no surgery (open circle) control.Grem1andLeprn= 4 animals/group,Acann= 3 animals/group. Paired, two-tailt-test.gColVII induced OA experiment schema.hRepresentative images ofGrem1-TdTdistal femur joints showing loss ofGrem1-lineage AC cells as indicated by arrows within the injury site (top), and OA pathology induced by ColVII compared to PBS control. Sections stained with Toluidine blue and Fast green, arrows indicate superficial lesions.iQuantification of the percentage ofGrem1-lineage AC cells per HPF (left) and, unblinded histopathological assessment using OARSI grading of OA pathology (right) in ColVII induced OA (square) compared to PBS controls (circle).n= 6 mice/group. Paired, two-tailedttest.jRepresentative images of TUNEL staining in articularGrem1-lineage cells quantified ink.kQuantification of the number of articularGrem1-lineage TUNEL positive cells in ColVII induced OA (square,n= 8 mice) compared to PBS control (circle,n= 7 mice). Unpaired, two-tailedttest. Bars denote s.e.m. Source data are provided as a Source Data file. Mouse image in figure schemas created with BioRender.com. 4f and Supplementary Table 1 ). Consistent with previous studies, this included enrichment of the AC marker, Lubricin ( Prg4 ), in AC compared to GP Grem1 -lineage cells [37] (Supplementary Fig. 4g ). Fig. 4: Grem1 -lineage single cell transcriptomics revealed a distinct population of articular chondrocytes that can be targeted for therapy. a Single cell RNA (scRNA) sequencing data showed distinct clusters of cells isolated from the AC and GP of Grem1-TdT mice compared to Lepr -lineage cells isolated from the Lepr-TdT mice. b Heat map depicting unsupervised clustering of top 10 differentially expressed transcripts between the different clusters in a . c Grem1 -lineage AC cells co-expressed genes important for AC function ( Foxo1 ) and receptor ( Fgfr3 ) for FGF18 treatment. One-sided chi-Square correlation analysis confirmed co-expression of Foxo1 and Fgfr3 in Grem1 expressing cells ( p = 0.00113). d Experiment schema. e Representative images of fluorescent Grem1 lineage tracing in the articular joint with or without Foxo1 deletion (top) with OA lesions highlighted using red arrows, and Toluidine blue and Fast green stain (bottom) with arrows indicating cartilage lesions and chondrocyte disorganisation. n = 5 animals per group. f Percentage of Grem1 -lineage ACs per HFP in control Grem1-TdT mice (circle) compared to Grem1-TdT-Foxo1 mice (square), n = 6 mice/group. g Unblinded histopathological OARSI scoring in Grem1-TdT-Foxo1 mice (square) compared to Grem1-TdT mice (circle), n = 5 mice/group. f , g bars denote st.dev. h Experimental schema. i Representative images of joints from Grem1 -lineage mice with ColVII induced OA with or without FGF18 treatment with arrows indicating injury site (fluorescence, top), toluidine blue and fast green stained showing proteoglycan loss and lesions indicated by arrows (bottom). j Quantification of the percentage of Grem1 -lineage cells with FGF18 treatment (left, n = 6 mice/group), OA score (middle, n = 6 mice/group) and AC thickness (right, n = 5 mice/group). Bars denote s.e.m. f – j unpaired, two-tailed t test. Source data are provided as a Source Data file. Mouse image in figure schemas created with BioRender.com. Full size image Immunofluorescence staining of tissue samples from 2 week lineage traced Grem1-TdT mice showed overlap between articular Greml -lineage CP and PRG4 expressing cells (12.6% of the articular cartilage double positive), but the Greml -lineage cells were largely distinct from COL2-expressing chondrocytes in the calcified zone (<0.1% articular cartilage cells double positive for Grem1 -lineage and COL2, Supplementary Fig. 4h ). Most Grem1 -lineage cells separately prepared from whole bone expressed the defining marker of mSSC, CD200 [15] (Supplementary Fig. 4i ), but only 19% of Grem1 -expressing cells from the articular surface had a transcriptomic profile consistent with the mSSC immunophenotype (Supplementary Fig. 4j, k ). This indicates that Grem1 -lineage CP in the articular surface and mSSC in the GP partially overlap, but the articular surface Grem1 -lineage population is distinct. Next, we investigated gene expression associated with cartilage development and regeneration across the scRNAseq data set. Forkhead box protein-o ( Foxo) genes have important roles in apoptosis, cell-cycle progression, resistance to oxidative-stress and maintenance of stem cell regenerative potential [38] , [39] . We observed that Foxo1 expression was highly correlated with Grem1 expression ( p < 0.0001) in articular CP cells in our scRNAseq data [40] (Fig. 4c ), with Foxo1 expression also significantly increased in the AC compared to GP Grem1 -lineage populations (Supplementary Fig. 5a ). At the protein level, the majority of FOXO1 expressing cells in the adult AC were Grem1 -lineage cells, while there were very few FOXO1 expressing Grem1 -lineage cells observed in the GP (Supplementary Fig. 5b ). To determine whether Foxo1 expression was essential for survival of Grem1 articular CP cells and prevention of OA, Grem1-TdT mice were crossed to Foxo1 fl/fl mice, to produce Grem1-TdT-Foxo1 conditional knock-out mice. Grem1-TdT-Foxo1 mice were administered tamoxifen at 6 weeks of age to induce Foxo1 deletion in Grem1 -lineage cells and sacrificed at 26 weeks (Fig. 4d ). Significantly fewer Grem1 -lineage AC but not GP cells were observed in Grem1-TdT-Foxo1 mice, in comparison to age-matched Grem1-TdT controls, and the resulting increased OA pathology resembled Grem1-creERT;DTR DT ablation (Fig. 4e–g , Supplementary Fig. 5c ). This suggested that Foxo1 was important to maintain adult Grem1 -lineage articular CP cells and, by extension, AC integrity. Interestingly, Grem1-TdT-Foxo1 mice administered tamoxifen in the early neonatal period (Day 4–6) developed drastic Grem1 -lineage articular CP cell loss, more severe OA pathology and decreased AC thickness, in comparison to age-matched Grem1-TdT controls and Grem1-TdT-Foxo1 animals induced with tamoxifen in early adulthood (Supplementary Fig. 5d, e ). This indicates the crucial role for Foxo1 in AC development of the Grem1 -lineage CP cell population, as well as in adult AC maintenance. To discover molecular targets in Grem1 -lineage articular CP cells for OA therapy, we focussed on fibroblast growth factor (FGF) signalling, given the role of this pathway in regulating chondrogenesis [41] . Fibroblast growth factor receptor 3 ( Fgfr3) was expressed both in Grem1 -lineage GP and articular CP populations. Aware of the important role for fibroblast growth factor 18 (FGF18) as a key agonist of FGFR3 as an experimental treatment for OA [42] , we investigated the impact of exogenous FGF18 on Grem1 -lineage AC stem cells in vivo. Adult Grem1-TdT mice induced with tamoxifen were injected intra-articularly with 0.5μg FGF18 or PBS twice weekly for 2 weeks and concurrently administered EdU to label newly proliferating cells (Supplementary Fig. 5f ). FGF18 treatment resulted in a significant increase in both the number of EdU+ Grem1 -lineage articular CP cells and AC thickness, suggesting FGF18 induces AC chondrogenesis in the adult knee via increased Grem1 -lineage articular CP cell proliferation (Supplementary Fig. 5g, h ). Notably, very few EdU+ cells were found in the hypertrophic chondrocyte zone, suggesting that the neo-cartilage arises from the articular CP population. To determine whether FGF18 can also rescue OA pathology, we used ColVII to induce OA and then intra-articularly injected Grem1-TdT mice with 0.5 μg FGF18 or PBS twice weekly for 2 weeks. FGF18 injection resulted in a significant increase in Grem1 -lineage CP cells and AC thickness in treated joints compared to PBS controls and a significant reduction in OA pathology (Fig. 4h–j and Supplementary Fig. 5i ). This suggested that exogenous FGF18 alleviates OA through increased Grem1 -lineage CP cell proliferation. OA, like other degenerative diseases, can be viewed as the dysfunction of mature cartilage cells or the result of an imbalance in stem-progenitor cell repair and renewal. Previous studies have shown functional cartilage cell dysfunction/death results in OA, here we show that ablation of a restricted progenitor population can cause OA without disturbing the broader population of differentiated chondrocytes. While stem cell therapy for OA using traditional MSC populations has shown promise in reducing pain and stiffness, it does not effectively repair normal AC [43] , [44] . Several research teams, including our own, have recently described SSCs with lineage potential restricted to cartilage, bone and stroma that are promising candidates for joint disease treatment [13] , [15] , [16] . 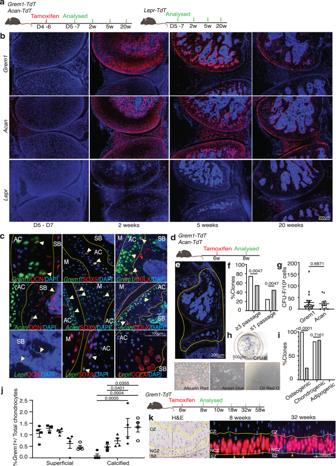Fig. 2:Grem1-lineage marks a progenitor cell population in the AC. aExperimental schema.bRepresentative images of AC fromGrem1-TdT(top row) andAcan-TdT(middle row) mice and age pairedLepr-TdT(bottom row) mice.n= 5 animals per group per time point.cDistal femur from neonatal tamoxifenGrem1-TdT,Acan-TdTandLepr-TdTpulse-chased for 20 weeks. Representative IF staining ofGrem1(top row),Acan(middle row) andLepr(bottom row) cells expressing OCN, SOX9 and COLX (indicated by yellow arrows). Subchondral bone (SB), articular cartilage (AC) and meniscus (M).n= 3 mice per group.dExperimental schema.eArticular joints, outlined in yellow, were used to isolate red cells for in vitro assays.fPercentage ofGrem1-lineage (white) clones able to undergo expansion compared toAcan-lineage (grey) clones.gNumber of CFU-F formed per clone.h, Representative images ofGrem1-lineage cells stained for CFU-F or differentiation markers Alizarin Red (osteo), Alcian blue (chondro) and Oil Red O (adipo).iNumber ofGrem1- (white) orAcan-lineage (grey) clones that had undergone differentiation quantified as % of the total number of clones.f–icells pooled fromn= 3 animals, 22 clones per lineage.jExperimental Schema (right). Quantification of the total number ofGrem1-lineage cells within the superficial and calcified zones as a percentage of the total number of chondrocytes within the AC at 8 weeks (filled circle,n= 4 mice), 10 weeks (square,n= 3 mice), 18 weeks (triangle,n= 4 mice), 32 weeks (diamond,n= 4 mice) and 58 weeks (open circle,n= 4 mice) of age (left). Bars show s.e.m.kRepresentative images of adult articular joint showing H&E of zonal organisation of chondrocytes in the superficial zone (SZ), non-calcified zone (NCZ) and calcified zone (CZ) andGrem1-lineage AC cells moving towards the CZ from 8 weeks (middle) to 32 weeks (right) of age. Superficial chondrocytes indicated with yellow arrows.f,iTwo-sided Fisher’s exact test.gTwo-sided unpairedttest.jTwo-way Anova Tukey’s test. Bars denote s.e.m. Source data are provided as a Source Data file. Mouse image in figure schemas created with BioRender.com. In this study, we show that Grem1 -lineage CP cells contribute to neonatal generation of the AC and are pivotal to AC maintenance in adulthood. In vitro, the articular Grem1 -lineage cells display clonogenicity and multi-potent differentiation properties associated with stemness, however, a complete assessment of their potential stem cell properties and lineage hierarchy using in vivo transplantation studies [15] , [45] remains to be undertaken. The position of adult Grem1 -lineage traced cells on the superficial surface of the AC, and subsequently in deeper layer chondrocytes and subchondral bone, is consistent with previous descriptions of chondrocytic label retaining progenitors and the Prg4 (encoding lubricin) lineage where tracing began from birth or in juvenile mice, not adults as investigated here [7] , [37] . A key difference between the Prg4 - and Grem1 -lineages is that Grem1 -expressing cells contribute to both articular and growth plate chondrocytes [37] . Although the AC and GP are both broadly constituted by chondrocytes, these structures form quite differently and have differing roles in skeletogenesis [46] , [47] , with the AC being the primary site of OA pathology. Our focus has been on the articular Grem1 -lineage population and superficial chondrocytes as this is the site of early OA-like changes. We cannot discount, however, that the GP Grem1 -lineage CP cells may also contribute to the articular phenotypes observed and have not categorically excluded that Grem1 -lineage subchondral bone populations may arise in part from GP resident progenitors. Equally, we have not investigated which Grem1 -lineage population gives rise to the meniscus or if the Grem1 promoter is independently active at sites throughout the knee joint. We show that some, but not all, acutely labelled Grem1 -lineage articular cells express Prg4 /PRG4 and/or Acan, and are distinct from the COL2-expressing chondrocytes of the calcified zone (Supplementary Fig. 3l , 4h ). Other key differences between the Grem1 -lineage and that of the broader chondrocytic population marked by Acan include the extent and location of labelled lineage cells (Fig. 2e , Supplementary Fig. 2b ), differential expression of cartilage-related transcripts (Supplementary Fig. 3n ), clonogenicity and differential potential ex vivo (Fig. 2d–i ) and response to injury (Fig. 1b–f ), such that Grem1 - but not Acan -lineage cells were lost in the early OA-like phenotype induced by DMM surgery. Ablation of Grem1 -lineage CP cells in the knee joint causes OA, with a milder phenotype observed using similar induction protocols and transgenic mouse models to ablate Acan -lineage cells (Supplementary Fig. 3k, o ). Likewise, as FOXO1 expression is restricted to the superficial chondrocytes of the AC (Supplementary Fig. 5b ), genetic deletion of Foxo1 in Grem1 -lineage cells effectively depletes FOXO1 expression in the articular surface, rather than deeper chondrocytic layers and results in OA. This suggests the Grem1 -expressing cells represent a specific subset of the total chondrocyte population that may be lost early in the disease process. We acknowledge that OA can be caused by dysfunction of mature cartilage cells, but here also highlight the importance of dysfunction and loss of a specific chondrocyte progenitor population marked by Grem1 . This is supported by phenotypic differences resulting from adult Prg4 and Grem1 -lineage ablation. Loss of both Prg4 - and Grem1 -lineage populations resulted in decreased superficial chondrocytes, however cartilage deterioration and OA histological features only occurred following loss of Grem1 -, and not Prg4 -, lineages [36] (Fig. 3 ). Similar to mSSC cells [13] , Grem1 -lineage articular CP cells are lost with age. Using two mouse models of OA, we found that Grem1 -lineage CP cells in the knee joint were lost in early injury. We also report that functional ablation of Grem1 -lineage articular CP cells, or genetic deletion of Foxo1 in Grem1 -lineage cells, in early adult mice led to significant and rapid OA (Figs. 3 , 4 ). As efforts to reintroduce Grem1 articular CP cells would be a natural first step to therapeutics, our initial efforts were not successful (Supplementary Fig. 3q ) and future efforts using a bio- scaffold with factors to stimulate enhanced chondrogenesis are warranted. scRNAseq analysis identified separate populations of Grem1 -lineage cells within the AC and GP structures, that provided an insight to the restricted commitment of each population of cells. FGF18 treatment induced proliferation of Grem1 -lineage articular CP cells and reduced OA pathology, presenting a strong candidate for further clinical trials of OA prevention and therapy for early disease. We propose that OA can be predisposed by inadequate reserves of, or injury to, articular CP cells (accompanied by the loss of surface proteoglycan and cartilage fibrillation), followed by the apoptotic death of further CP cells, and the resulting failure to regenerate articular cartilage. This study reframes OA as a cellular disease that can result from CP cell loss and provides a biological focus for OA therapy. Mice LepR-cre [48] , Acan-creERT [49] , Grem1-creERT [16] , R26-LSL-TdTomato [50] , R26-LSL-ZsGreen [50] and R26-LSL-iDTR were imported from Jackson Laboratory and bred within the South Australia Health and Medical Research Institute (SAHMRI) Bioresources facility and Institute of Comparative Medicine at Columbia University. Grem1-TdTomato-iDTR mice ( Grem1-creERT;DTR) were generated by mating homozygous Grem1-TdT mice to homozygous Rosa-iDTR . Acan-iDTR mice ( Acan-creERT;DTR) were generated by mating heterozygous Acan-creERT mice to homozygous or heterozygous Rosa-iDTR . All animal experiments complied with all relevant ethical regulations and were approved by the Animal Ethics Committee at the SAHMRI under ethics number SAM189 and SAM385.19 and at Columbia University. Mice were maintained in the South Australia Health and Medical Research Institute (SAHMRI) Bioresources facility and Institute of Comparative Medicine at Columbia University, in accordance with JAX USA animal husbandry protocols. Animals were given food and water ad libitum and housed in temperature- (average 21–22 °C), moisture-(45–55% humidity), and light-controlled (12 h light/dark cycle) individually ventilated cage systems. 10–13 weeks old Grem1-TdT, Acan-TdT, LepR-TdT and C57BL/6 male mice were used to examine lineage tracing in health and DMM surgery model. Postnatal Day 4–6 (neonatal) and 6 weeks old (adult) Grem1-TdT, Acan-TdT and LepR-TdT mice were used to examine lineage tracing in early development and adulthood. 8 weeks old Grem1-TdT mice were given tamoxifen at 6 weeks of age to examine in vitro stem cell properties. 26-week-old Grem1-creERT;FOXO1 mice were given tamoxifen at postnatal Day 4–6 (neonatal) and 6 weeks of age (adult) to examine the AC impact of FOXO1 deletion in Grem1 cells. 5–6 week old Grem1-TdT mice were given tamoxifen for ten days, then harvested at 7–9 weeks of age for scRNAseq analyses. 4–6 week old Grem1-TdT mice were used to examine the treatment of Fgf18 in AC with or without CiOA 4–6 week old Grem1-TdT mice were used to examine the treatment of Fgf18 in AC with or without CiOA. 4–7 week old Grem1-Td-DTR , Grem1-creERT;DTR and Acan-creERT;DTR mice were used to examine the impact of the ablation of Grem1 -lineage and Acan -lineage cells on AC. Generation of knock-in Grem1 -DTR-TdT mice by CRISPR/Cas9 mediated genome engineering To generate a DNA construct for Diphtheria Toxin Receptor (DTR) / tdTomato (tdTom) expression under the control of the endogenous Grem1 promoter in mice, we first used gene synthesis to insert the coding sequence for DTR immediately downstream of a 2 A peptide from porcine teschovirus-1 polyprotein (P2A), followed by a second P2A sequence and the coding sequence for tdTom, all within two exon2 2 kb Grem1 homology arms (Supplementary Fig. 6 ). The construct was Sanger sequence verified (Geneuniversal) and used for subsequent gene targeting in mice. C57BL6/J female mice were superovulated with 5 IU Pregnant Mare Serum Gonadotrophin (PMSG; Folligon; Intervet) and 47.5 h later with 5 IU human chorionic gonadotrophin (hCG; Chorulon; Intervet) before being mated to C57BL6/J males. Presumptive zygotes were collected from oviducts 19 h post-hCG injection in FHM media (Merk Millipore) and maintained in KSOMAA media (Merk Millipore) under oil at 37 °C in 5% CO 2 5% O 2 with a Nitrogen balance. Fertilized zygotes were identified in FHM media under oil by the presence of two pronuclei before microinjection of 25 ng/ul SpCas9 protein (PNA Bio), and 10 ng/ul SpCas9 single guide RNA (sgRNA) (CGACTTGGATTAAGTCAAAG) with the donor plasmid at 10 ng/ul, in a buffered solution. Genomic DNA was isolated from ear notches using a High Pure PCR Template Preparation Kit (Roche) and Knock-in (KI) founder screening was performed using a forward primer (GCCTGGGATATTCTGAGCCC) and a reverse primer (GTCCCGCGCATTTTGACTTT). KI allele in the founder mouse was confirmed by PCR and Sanger sequencing across the entire locus from outside of the donor homology arms before mating with C57BL6/J to create second generation line. Tamoxifen administration Neonatal Grem1-TdT and Acan-TdT mice were subcutaneously administered 2 mg tamoxifen (#T5648, Sigma) dissolved in peanut oil at Day 4–6 of age for lineage tracing studies. Grem1-TdT and Acan-TdT adult lineage tracing mice were administered 4 doses of 6 mg tamoxifen dissolved in peanut oil via oral gavage at ages specified in figures. Grem1-TdT and Acan-TdT DMM OA mice were administered 4 doses of 6 mg tamoxifen dissolved in peanut oil via oral gavage at 8–10 weeks of age. Grem1-TdT ColVII OA and Grem1-creERT;DTR mice were administered 5 separate doses of 4 mg tamoxifen via daily oral gavage over 9 days (1 day off dosing in between) from 6 or 4 weeks of age, respectively. EdU labelling of Grem1-TdT mice was performed by administering 5 separate doses of 4 mg tamoxifen via daily oral gavage over 9 days and commenced on EdU in drinking water 2 weeks prior to collection. Grem1-TdT mice for scRNA experiments and ACAN co-immunofluorescence staining were administered 500 mg/kg tamoxifen chow for 10–14 days from 5–6 weeks of age. Diphtheria toxin (DT) administration Grem1 cells within the AC are abundant at 2 weeks of age, therefore, we selected mice at this age for initial validation of Grem1 cell ablation within the AC. Diphtheria toxin (#BML-G135, Enzo) at a concentration of 250 ng in 10 µL of PBS was injected intraperitoneally into 2-week-old Grem1-Td-DTR and mice sacrificed 2 days later. Anti-RFP immunohistological staining was performed to validate the distribution and ablation of Grem1 cells in the Grem1-Td-DTR AC compared to aged matched Grem1-TdT mice (Supplementary Fig. 3g ). For OA pathology, mice 5–7 weeks of age were administered two doses of 250 ng DT intra-articularly in 10 µL of PBS and limbs collected 3 days later for analysis and blinded scoring of OA pathology. Grem1-Td-DTR mice administered with DT developed a fatal small intestinal phenotype at day 4 for homozygous mice and at day 7 for heterozygous mice after DT injection. A similar phenotype has been previously reported [51] . Ablation of Grem1 -lineage cells in Grem1-creERT;DTR mice and Acan -lineage cells in Acan-creERT;DTR mice was performed by administering 100–125 ng of DT (#D0564, Sigma) intra-articularly 3 times weekly for 2 weeks into 8 week old mice that were given tamoxifen prior at 4–6 weeks of age. Mice were then sacrificed at 26 weeks of age for analysis and unblinded OARSI scoring. Destabilisation of the medial meniscus surgery (DMM) DMM surgery was conducted using an established protocol [52] approved by the SAHMRI Bioresources Animal Ethics Committee. Briefly, surgery was performed on male mice between the ages of 10–13 weeks that had previously been administered tamoxifen. Animals underwent general anaesthesia via isoflurane inhalation. The right hind limb of the animal was shaved with a razor blade to provide a clean surface and left hind limb was used as a paired normal control. Skin incision was made on the medial side of the patella, using sterile scissors, to expose the patella. Once the patella was exposed, a second incision was made on the medial side and the incision site was extended so that the patella could be luxated. Using sterile gauze, the fat pad located on the knee was pushed aside to expose the medial meniscotibial ligament, the ligament was then transacted using a twisting motion. Bleeding was controlled throughout surgery, and the cartilage was kept moist with sterile saline. The patella was then repositioned back, and the incision sites and patella were sutured. Collagenase VII induction of OA (CiOA) The collagenase-induced OA model involves intra-articular injection of Type VII Collagenase as described [22] . Briefly, 8-week-old mice previously administered with tamoxifen were injected intra-articularly with 10 µL of 2U ColVII (#C0773, Sigma-Aldrich) dissolved in PBS under a dissection microscope. Histology Mice were humanely sacrificed, bones from both hind limbs were collected and all muscles removed before fixing in 4% paraformaldehyde overnight, decalcified in Osteosoft® (#101728, Millipore) for 3–10 days and dehydrated in 30% sucrose at 4 °C before embedding in OCT compound (Sakura Tissue-Tek). Embedded tissues were stored at −80 °C. 10 μm frozen sections were collected on cryofilm (type IIC(10), Section-Lab) for staining. 0.04% toluidine blue (#198161, Sigma) in 0.1 M sodium acetate pH4.0 or 0.1% Safranin O (#8884, Sigma) in water, and 0.1% fast green (#F7252, Sigma) stain in MilliQ water was used to demonstrate histological features of cartilage and bone. Haematoxylin and eosin (H&E) staining of the AC region was used to identify different organisational zones within the adult AC. Quantification of cells and AC thickness Lineage-traced ( TdTomato positive) cells within the AC were counted throughout the femur and represented as a percentage of the total number of chondrocytes (DAPI positive). Only TdTomato cells colocalised with DAPI were included to avoid the inclusion of dead cells. AC cells in neonatal tracing were defined by the thin and highly cellular structures consisting of small and closely bound cells. Serial sections stained with H&E were used to guide the zonal separation of the AC. Cells in both the femur and tibia AC in 3 randomly selected images at 40x magnification per sample were used to quantify the number of lineage-traced cells per high power field (HPF) and represented as a percentage of the total number of chondrocytes. AC thickness was measured by averaging 3 randomly selected areas of the AC in the femur and tibia. Final AC thickness was represented as an average of 3 slides per sample. EdU and TUNEL positive Grem1 -lineage cells were quantified in 3 randomly selected images at 40x magnification per sample and represented as total number of positive cells per HPF. Only EdU positive cells within 1-4 cells from the superficial zone of the articular layer were counted. OA pathology scoring OA pathology (both femoral and tibial) in Grem1-creERT;DTR mice were scored using histological sections in an unblinded fashion using the 0–6 OARSI scoring system [23] . Final OARSI scores represent the average of 3 slides per sample. OA pathology in the Grem1-TdT-DTR experiments were scored blinded using scoring parameters of AC damage (0–11), proteoglycan loss (0–5), chondrocyte hypertrophy (0–3), subchondral bone sclerosis and vascular invasion (both 0–3), osteocyte size and maturity (both 0–3) and meniscus pathology (0–20) as described [53] . The average scores of 2–3 slides per sample, total of 8 parameters, were summed to produce the final score. The average OA scores of both tibia and femora were included in this study. Immunohistological and fluorescent staining Immunohistochemistry and immunofluorescent staining were completed on 10μm frozen sections. Antigen retrieval was performed by placing slides in a steamer submerged in antigen unmasking solution (#H-3300, VectorLab) for 6 min. 0.025% v/v triton X-100 in PBS was used for anti-RFP staining. Immunohistochemistry slides were treated for endogenous peroxidase activity by incubating in 3% H 2 O 2 for 30 min. Blocking was performed in 2% BSA, 5% normal goat and 5% normal donkey serum. The following antibodies were used: anti-PCNA (#ab18197 Abcam, 1:200), ColX (#ab58632 Abcam 1:200), OCN (#ab93876 Abcam, 1:200), Lubricin/PRG4 (#ab28484 Abcam, 1:250), COL2 (#ab34712 Abcam, 1:250), FOXO1 (#MA5-32114 ThermoFisher Invitrogen, 1:150), Sox9 (#AB5535 Millipore, 1:400), ACAN (#AB1031 Merck Millipore, 1:100) and anti-RFP (#600-401-379, Rockland 1:250). After overnight incubation at 4 °C, slides were washed with PBST and incubated with species-appropriate secondary antibody (1:200–1:300) at room temperature for 1 h. Finally, slides were counter stained with DAPI before mounted with a cover slip. For immunohistochemistry, after overnight incubation at 4 °C, slides were washed with PBST and incubated with anti-rabbit biotin (#BA-1000, VectorLab 1:250) at room temperature for 1 h and then streptavidin-HRP (#SA-5004, VectorLab 1:100) at room temperature for 30 min and developed with DAB chromogen (#K3468, Dako). EdU staining was done using the Click-iT EdU proliferation kit (#C10086, ThermoFisher) as per manufacturer’s instructions. Imaging Stained sections were scanned using the 3DHistech Panoramic 250 Flash II to generate brightfield images. Fluorescent images were captured either on a Olympus IX53 and Nikon Eclipse Ti inverted microscope or the Leica TCS SP8X/MP confocal microscope. Images of whole bone were achieved by stitching together 20–24 images at 10x magnification using ImageJ software. Grem1 Chondroprogenitor Cell isolation Both hind limb bones (femur and tibia) were collected from 8-week-old mice that had been subjected to tamoxifen and all muscles and ligaments removed. To limit contamination from non-articular cell populations present in whole bone preparations, the knee joints were dislocated at the epiphyses from both femur and tibia to exclude the GP-cartilage, gently disrupted using a mortar and pestle, and digested in 4 mg/ml collagenase IV (#17104019, Gibco) and 3 mg/ml Dispase (#17105041, Gibco) in α-MEM (#M5650, Sigma). Collected cells were then sorted for lineage-traced articular TdTomato positive cells. Cells were sorted based on forward and side scatter, single cells as well as positive for TdTomato fluorescence. Live and dead (DAPI) staining was omitted to allow for later expansion of clones in DAPI free conditions. Sorted cells were plated in complete media (α-MEM supplemented with 20% defined bovine serum, 100 mM L-ascorbate-2-phosphate, 1 mM sodium pyruvate, 50 μg/ml streptomycin, 50 U/ml penicillin, 2 mM L-glutamine and 10μM Y-27632) at 1000 cells per 10 cm dish to allow for isolation of individual clones using clonal cylinders (#Z370789, Sigma). A total of 22–24 clones (i.e., isolated adherent clusters of >50 cells at 10–14 days) were harvested and allowed to expand before performing clonogenicity and multilineage differentiation assays. Both clones that expanded and did not expand were collected for qPCR analysis. Clonogenicity and multilineage differentiation Colony-forming unit—fibroblasts (CFU-F) assay was performed by seeding cells at clonal density (1000 cells per 10 cm dish) and subsequently cultured in complete media for 14 days. The cultures were stained with 0.1%w/v toluidine blue in 2.4% formalin solution and the total number of colonies counted, where an individual colony was defined as ≥50 cells. The number of clones was reported as (CFU-F)/1000 cells plated. Induction of osteogenic, chondrogenic and adipogenic differentiation was conducted by maintenance of cell cultures in differentiation media (StemPro) as per manufacturer’s instructions. Positive and negative assessment of differentiation potential was performed by staining cells with 2% w/v Alizarin red in water pH 4 (osteogenesis), 0.1% w/v Alcian blue in 0.1 N HCl (chondrogenesis) and 0.5% w/v Oil Red O in isopropanol diluted further in a 6:4 ratio in water (adipogenesis). All in-vitro assays reported in this study were conducted on clonal cell populations of passage 5 or lower. RNA isolation and RT-PCR Total RNA was isolated from cells using TRIzol (Thermofisher) as per manufacturer’s instructions. Complementary DNA (cDNA) was generated using SuperScript IV reverse transcriptase kit (Invitrogen) according to manufacturer’s protocol. Transcript levels were assessed by QuantStudio 7 (Thermofisher) using IDT probes GAPDH (Mm.PT.39a.1) and Grem1 (Mm.PT.53a.31803129) with the FastStart TaqMan Probe Master (#04673409001, Roche). Flow Cytometry for assessment of mSSC markers in Grem1 -lineage cells All limbs were collected from 8-week-old mice that had been subjected to tamoxifen and all muscles and ligaments removed. Cleaned bones (i.e., whole bone preparation) were gently disrupted using a mortar and pestle, minced, and digested in 2.5 mg/mL collagenase I (#CLS-1, Worthington). Collected cells were subjected to RBC lysis and blocked with 3% BSA, 2% FCS in PBS. The following antibodies were used: anti-CD45 (#103131, BioLegend, 1:80), anti-Ter119 (#116227, BioLegend, 1:80), anti-CD31 (#562861, BD Pharmingen, 1:80), anti-CD200 (#ab33735, Abcam, 1:10), APC/Cy7 Streptavidin (#405208, BioLegend, 1:300) and DAPI (#D9542, Sigma-Aldrich). Cells were sorted on FACSFusion or LSR Fortessa (BD Biosciences) based on forward and side scatter plots, single cells, live cells (DAPI negative), trilineage expression (CD45 - Ter119 - CD31 - ) and lineage reporter positive fluorescence. Single cell sorting for scRNAseq analysis Grem1-TdT mice at 5–6 weeks of age were subjected to tamoxifen chow for 10–14 days before they were sacrificed. Age paired LepR-TdT mice were used for the analysis presented in Fig. 4 . Hind limbs were collected, and all muscles and ligaments removed. AC alone (Fig. 3 ), or AC and GP (Fig. 4 ) from Grem1-TdT mice were separately excised under a dissection microscope and kept as separate tissue samples (AC and GP) through subsequent mincing using a scalpel before being digested in 2.5 mg/mL collagenase type II (#CLS-2, Worthington). Cleaned LepR-TdT whole bones were gently disrupted using a mortar and pestle, minced, and digested in 2.5 mg/mL collagenase type I (#CLS-1, Worthington). The following antibodies were used: anti-CD45 (#103111, BioLegend), anti-Ter119 (#116211, BioLegend), anti-CD31 (#102509, BioLegend), and DAPI (#D9542, Sigma-Aldrich). LepR cells were sorted based on forward and side scatter, single cells, live cells (DAPI negative), trilineage negative expression (CD45-Ter119-CD31-) and TdTomato positive fluorescence. Grem1 cells from the AC or GP (GP Fig. 4 only) were sorted separately based on forward and side scatter, single cells, live cells (DAPI negative), and TdTomato positive fluorescence, to generate separate Grem1 -lineage populations derived from the AC (or GP). Individual cells were randomly allocated into 96-well plates to avoid batch effects, in lysis buffer previously prepared by the Sulzberger Genome Centre (Columbia University, Fig. 4 ) or encapsulated in Gel Beads-in-emulsion (GEMs) using a Chromium Controller (10× Genomics, Pleasanton, CA, USA, Fig. 3 ). Library preparation was performed using Chromium Single Cell 3’ Library & Gel Bead Kit v3 (10× Genomics, Pleasanton, CA, USA) following the manufacturer’s protocol and sequenced using Illumina NextSeq 500 at Columbia University Genome Centre’s Single Cell Analysis Core. Single cell sequencing analysis Raw Illumina data were processed to convert Illumina basecall files to FASTQ format. Alignment of reads to the mouse genome (mm10) version 2020-A and gene counting was performed using the 10× Genomics Cell Ranger pipeline (10× Genomics, Pleasanton, CA, USA). Cells from 2–3 individual samples were grouped together. Count tables were analysed in the R environment (version 4.0.2 or 4.3.1) with the Seurat package (version 3.2.2 or v5). Figures 3 and 4 experiments and analyses were undertaken separately with analyses as follows. 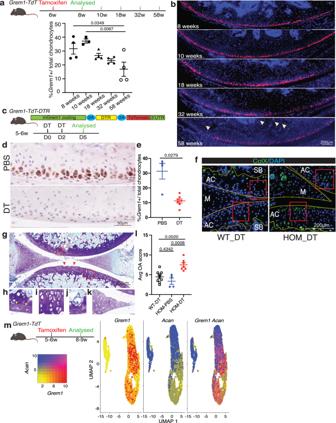Fig. 3:Grem1-lineage articular progenitors cells are lost with age and targeted ablation causes OA. aExperimental schema. Quantification of totalGrem1-lineage articular chondrocytes (AC) as a % of the total ACs.n= 4 animals per time point, except 10wkn= 3. One-way Anova Tukey’s test.bRepresentative images of theGrem1-TdTarticular knee joint froma.cSchematic of theGrem1-Td-DTRknock-in construct (top) and experimental outline.dRepresentative images of early adult mice articular joints treated with PBS or DT stained with anti-RFP.eQuantification ofGrem1AC cells as a % of the total number of AC chondrocytes in PBS (blue,n= 4 mice) or DT treated (red,n= 7 mice)Grem1-Td-DTRmice. Two-tailed Welch’sttest.fRepresentative images of ColX staining ofGrem1-Td-DTRjoints from WT and HOM DT-treated animals,n= 3 mice/group. Boxed regions indicate loss of ColX chondrocytes following ablation ofGrem1-expressing articular cells in HOM DT treated mice.gRepresentative image of DT treated articular joint ofGrem1-Td-DTRmice (n= 7 mice) stained with Tol blue and fast green showing pathological changes commonly associated with OA including AC damage indicated by red arrows,hloss of proteoglycan in the AC indicated by yellow arrows,ihypertrophic chondrocytes,jSB invasion, andkmeniscus pathology.lBlinded scoring of average OA score following 3 days DT treatment in control wild-type mice (WT-DT,n= 9 mice), homozygousGrem1-Td-DTRmice (HOM-DT,n= 7) or PBSGrem1-Td-DTRmice (HOM-PBS,n= 4). One-way Anova Tukey’s test.mSingle cell RNA (scRNA) sequencing experiment schema for isolation ofGrem1-lineage articular cells from mouse knee and analysis to show highGrem1 (red), highAcan(blue) or high bothGrem1/Acanexpressing (magenta) populations. Bars denote s.e.m. Source data are provided as a Source Data file. Mouse image in figure schemas created with BioRender.com. Figure 3 : Cells with fewer than 350 detected genes or genes that were expressed by fewer than 5 cells were excluded from the analysis. Dead cells and doublets were also removed by excluding cells that had more than 5% reads derived from mitochondria and cells with >5000 features. After removing all the unwanted cells from the dataset, the data was normalised by employing a global-scaling normalisation method ‘LogNormalize’. Subsequently, the 2000 most variable genes were identified, the data were scaled, and the dimensionality of the data was reduced by principal component analysis (PCA). A K-nearest-neighbour (KNN) graph based on the Euclidean distance in PCA space was constructed using the ‘FindNeighbors’ function and applied Louvain algorithm to iteratively group cells together by the ‘FindClusters’ function. A non-linear dimensional reduction was then performed via uniform manifold approximation and projection (UMAP) and various cell clusters were identified using a resolution of 0.6. Marker genes per cluster were calculated using Seurat’s ‘FindAllMarkers’ function and the ‘wilcox’ test option. To identify cells that express Acan and Grem1 , a subset of cells were extracted based on normalised and transformed expression of Grem1 and Acan with positive cells showing expression >0.25 and negative cells showing <0.25. Significantly differentially expressed genes between Grem1-/Acan+ and Grem1 + /Acan- cells were identified using Seurat’s ‘FindMarkers’ function and the ‘wilcox’ test option. 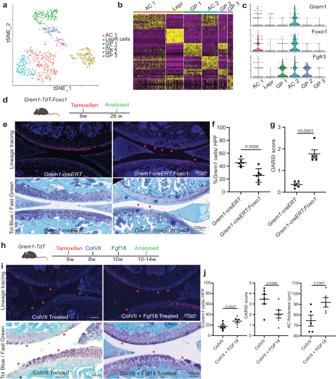Fig. 4:Grem1-lineage single cell transcriptomics revealed a distinct population of articular chondrocytes that can be targeted for therapy. aSingle cell RNA (scRNA) sequencing data showed distinct clusters of cells isolated from the AC and GP ofGrem1-TdTmice compared toLepr-lineage cells isolated from theLepr-TdTmice.bHeat map depicting unsupervised clustering of top 10 differentially expressed transcripts between the different clusters ina.cGrem1-lineage AC cells co-expressed genes important for AC function (Foxo1) and receptor (Fgfr3) for FGF18 treatment. One-sided chi-Square correlation analysis confirmed co-expression ofFoxo1andFgfr3inGrem1expressing cells (p= 0.00113).dExperiment schema.eRepresentative images of fluorescentGrem1lineage tracing in the articular joint with or withoutFoxo1deletion (top) with OA lesions highlighted using red arrows, and Toluidine blue and Fast green stain (bottom) with arrows indicating cartilage lesions and chondrocyte disorganisation.n= 5 animals per group.fPercentage ofGrem1-lineage ACs per HFP in controlGrem1-TdTmice (circle) compared toGrem1-TdT-Foxo1mice (square),n= 6 mice/group.gUnblinded histopathological OARSI scoring inGrem1-TdT-Foxo1mice (square) compared toGrem1-TdTmice (circle),n= 5 mice/group.f,gbars denote st.dev.hExperimental schema.iRepresentative images of joints fromGrem1-lineage mice with ColVII induced OA with or without FGF18 treatment with arrows indicating injury site (fluorescence, top), toluidine blue and fast green stained showing proteoglycan loss and lesions indicated by arrows (bottom).jQuantification of the percentage ofGrem1-lineage cells with FGF18 treatment (left,n= 6 mice/group), OA score (middle,n= 6 mice/group) and AC thickness (right,n= 5 mice/group). Bars denote s.e.m.f–junpaired, two-tailedttest. Source data are provided as a Source Data file. Mouse image in figure schemas created with BioRender.com. Figure 4 : all lineage traced cells were combined into one single cell object. When using FindClusters() function, dimensions of reduction were set from 1 to 9 and resolution was set at 0.6 to capture the majority of variation in the data (Supplementary Fig. 4c ). This unsupervised clustering identified 6 distinct cell clusters. We undertook quality control assessments to check that sequencing depth (indicated by unique molecular identifiers per cell), sample quality (mitochondrial and ribosomal content per cell) and proliferation markers were not drivers of cluster identity (Supplementary Fig. 4d ). Of the Grem1 -lineage cells, AC cluster 1(AC1) showed differential expression of a cytoprotective marker, Clusterin [54] , and early chondrogenic differentiation marker, Integral membrane protein 2A [55] ; AC cluster 2 (AC2) the hypertrophic chondrocyte marker Col10a1 [56] and early chondrocyte marker Sox9 [57] ; GP cluster 1 (GP1) and 2 (GP2) the cartilage angiostatic factor Chrondromodulin-1 (Cnmd) , known for its role in endochondral ossification and bone formation [58] , [59] , melanoma inhibitory factor ( Mia ) [60] and Matn3 which encodes an ECM protein that regulates cartilage development and homeostasis [61] while GP1 also expressed cartilage differentiation marker Serpina1 [62] ; GP cluster 3 (GP3) expressed cartilage degeneration marker Mmp13 [63] (Fig. 4a, b ). To explore single cell clusters that co-express Grem1 , Foxo1 and Fgfr3 a g ene count greater than 0 was used to define positive expression, and Chi-Square statistics were employed. For cluster analysis, FindAllMarkers() was used to generate marker lists, with parameters of min.pct = 0.25, logfc.threshold = 0.25, and tes.use = ‘roc’. To investigate the relationship between Grem1 AC cells with previously published mouse skeletal stem cells [15] (mSSCs; AlphaV + CD200 + CD45 − 6C3 − CD105 − Ter-119 − Tie2 − Thy − ), expression of the following combination of transcripts was investigated in the Grem1 AC population. Expression of Itga5 (encoding AlphaV) and Cd200 (encoding CD200) and lack of expression of Ptprc (encoding CD45), Enpep (encoding 6C3), and Eng (encoding CD105). Transcripts for Ly76 (encoding Ter119), Tek (encoding Tie2) and Thy1 (encoding Thy1.1/Thy1.2), were not detected in the AC populations and so were not included in the mSSC transcriptomic selection criteria. All violin plots were generated with VlnPlot() function in Seurat package and Chi-Square tests were performed with chisq.test() function in the base package. Statistical analysis All analyses were performed using Prism 8/9 (GraphPad Software Inc.), individual test details are provided in Figure legends. Line in dot plots indicate mean. Reporting summary Further information on research design is available in the Nature Portfolio Reporting Summary linked to this article.